Role of RIM1α in short- and long-term synaptic plasticity at cerebellar parallel fibres The presynaptic terminals of synaptic connections are composed of a complex network of interacting proteins that collectively ensure proper synaptic transmission and plasticity characteristics. The key components of this network are the members of the RIM protein family. Here we show that RIM1α can influence short-term plasticity at cerebellar parallel-fibre synapses. We demonstrate that the loss of a single RIM isoform, RIM1α, leads to reduced calcium influx in cerebellar granule cell terminals, decreased release probability and consequently an enhanced short-term facilitation. In contrast, we find that presynaptic long-term plasticity is fully intact in the absence of RIM1α, arguing against its necessary role in the expression of this important process. Our data argue for a universal role of RIM1α in setting release probability via interaction with voltage-dependent calcium channels at different connections instead of synapse-specific functions. The plasticity of synaptic connections is a core feature of neuronal networks that can be divided into short-term plasticity (STP, ms to s) and long-term plasticity (LTP, min to h) depending on duration. The molecular composition of synapses is critically important in determining STP and LTP, and generally the underlying cellular and molecular mechanisms are different. STP acts on synaptic connections between neurons on a fast time scale and the underlying events are for the most part taking place on the presynaptic side of a connection [1] . The direction of STP at a given synapse—that is, depression or facilitation—depends mostly on the initial release probability ( P r ) of a given synapse [2] . Among the factors that influence the P r are: the number of vesicles in the releasable pool, the number and type of voltage-dependent calcium channels (VDCCs), the spacing between the VDCCs and synaptic vesicles as well as the specific proteins mediating the priming and calcium sensitivity of release [3] . For the majority of synapses, LTP is both induced as well as expressed on the postsynaptic side [4] , ultimately leading to an alteration in AMPA receptor number or function. In contrast, only a rather specialized set of synapses displays presynaptic induction and expression of LTP, in which the synapses are finally strengthened through an increase in presynaptic transmitter release most likely involving changes at the release machinery [5] . Examples for this presynaptic type of LTP can be found in hippocampal mossy fibres [6] , cerebellar parallel fibres (PF) [7] and corticolateral amygdala synapses [8] as well as the subiculum [9] . Rab3-interacting molecule (RIM)1α is a presynaptically expressed protein of the active zone that has a key role in the docking and priming of synaptic vesicles [10] . It has also been implicated to be of great importance in both presynaptic STP and LTP. Remarkably, RIM1α was shown to be essential for LTP but not for STP at some connections (hippocampal mossy fibre and cerebellar PF synapses [11] , as well as hippocampal GABAergic synapses [12] ). In contrast, it was necessary for STP but not for LTP at the hippocampal Schaffer-collateral synapses [13] . The RIM interaction partner Rab3 displays a similar phenotype in that it influences STP at the hippocampal pyramidal neurons [14] , [15] and LTP, but not STP, at the mossy fibre synapses [16] . Therefore, synapses that show presynaptic LTP seem to rely on RIM1α for the expression, but STP at these connections remains unaffected by RIM1α loss. On the other hand, synaptic connections that obviously do not need RIM1α for LTP expression because of its postsynaptic origin do show altered STP without RIM1α. The only exception to this scheme described so far is the cortico-amygdala synapse where both presynaptic LTP as well as STP are affected by RIM1α loss [17] . More recently, the detailed mechanism how RIM operates was elegantly demonstrated at the calyx of Held [18] and in hippocampal cell cultures [19] , [20] using RIM1/2-conditional knockout (KO) mice. Those studies demonstrated that RIM assists in targeting calcium channels to active zones. RIM deletion resulted in a reduction in calcium current density at the calyx as well as a reduction in action potential-driven calcium transients in presynaptic boutons of the hippocampal pyramidal neurons. RIM was also shown to be important for the establishment of the size of the readily releasable pool and priming of synaptic vesicles. As a consequence of all the aforementioned effects, the P r is reduced in the absence of RIM, albeit only slightly, nevertheless leading to reduced short-term depression at the calyx of Held. For presynaptic LTP, the general consensus holds that a rise in presynaptic terminal calcium is necessary for induction [5] , [21] , [22] . Therefore, a subsequent question is, considering the interaction of RIM with VDCCs, whether the loss of RIM1α may lead to a failure of presynaptic LTP induction rather than having a role in LTP expression. In this report, we show that the deletion of a single RIM isoform, RIM1α, already causes a detectable phenotype at the cerebellar PF synapses in the form of reduced calcium influx leading to a reduced P r and consequentially an increased short-term facilitation. Moreover, we demonstrate here that despite the absence of RIM1α, long-term potentiation can be normally induced and expressed. Our data argue therefore for a universal role of RIM1α in setting the P r of synapses but do not support an indispensable function for presynaptic LTP expression. Enhanced short-term facilitation For this study we chose to investigate the cerebellar PF synapse—in this particular case meaning the connection of granule cells on Purkinje neurons. In a first set of experiments, we determined the properties of STP in the absence of RIM1α by recording from slices from genetic deletion mice. All numerical data are provided as ±s.e.m. We found a significant enhancement of paired-pulse facilitation of excitatory postsynaptic potentials (EPSCs) recorded from Purkinje neurons in RIM1α (−/−) mice compared with the control ( Fig. 1a , PPR for 50-ms ISI, WT: 1.76±0.05, n =14 cells, four mice versus KO 1.92±0.05, n =16 cells; six mice; P =0.036, Student’s t -test). We next applied a train of stimuli, consisting of 25 pulses delivered at 14 Hz, and also observed a considerably greater response over the whole time course of the train in KO mice ( Fig. 1b ; average of twenty first to twenty fifth pulses, WT: 1.4±0.09, n =10 cells, four mice versus KO: 1.9±0.1, n =11 cells, three mice; P =0.002, Student’s t -test, values normalized with respect to the first pulse in the train). These data demonstrate an enhanced short-term facilitation in the absence of RIM1α. 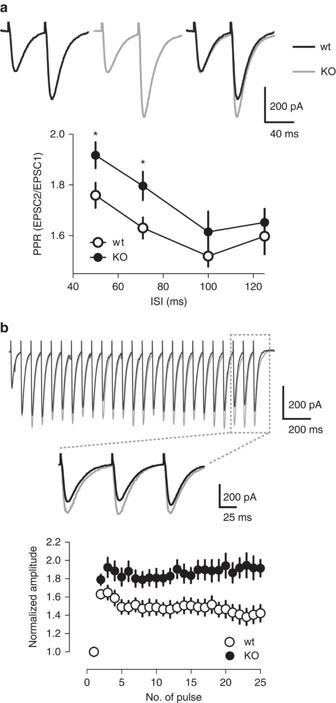Figure 1: Increased short-term plasticity in RIM1αknockout mice. Short-term facilitation was assessed by paired-pulse and train stimulation. (a) Paired pulses were applied with an interstimulus interval (ISI) of 50, 71, 100 and 125 ms. Representative traces (top) are shown for an ISI of 50 ms. Summary graph (bottom) for all ISIs, wild type (open circles) and knockout (filled circles); ISI 50 ms: n(WT)=14, n(KO)=16; ISI 71 ms: n(WT)=10, n(KO)=11; data points denote mean±s.e.m. *P<0.05, Student'st-test. (b) A 14-Hz train was applied for 25 pulses. Example traces (top) and summary plot (bottom) are shown; n(WT)=10, n (KO)=11, data report mean±s.e.m. The first two train pulses in (b) correspond to the 71-ms ISI in (a). The inset shows the last three responses in the train on an expanded time scale. Figure 1: Increased short-term plasticity in RIM1 α knockout mice. Short-term facilitation was assessed by paired-pulse and train stimulation. ( a ) Paired pulses were applied with an interstimulus interval (ISI) of 50, 71, 100 and 125 ms. Representative traces (top) are shown for an ISI of 50 ms. Summary graph (bottom) for all ISIs, wild type (open circles) and knockout (filled circles); ISI 50 ms: n(WT)=14, n(KO)=16; ISI 71 ms: n(WT)=10, n(KO)=11; data points denote mean±s.e.m. * P <0.05, Student's t -test. ( b ) A 14-Hz train was applied for 25 pulses. Example traces (top) and summary plot (bottom) are shown; n(WT)=10, n (KO)=11, data report mean±s.e.m. The first two train pulses in ( b ) correspond to the 71-ms ISI in ( a ). The inset shows the last three responses in the train on an expanded time scale. Full size image Reduced P r We then wanted to test whether the increased short-term facilitation might be caused by an alteration in P r because of the loss of RIM1α. For this purpose we performed two sets of experiments. In the first series, we made use of the competitive low affinity AMPA receptor antagonist γ- D -glutamylglycine (γDGG) (1 mM). We indeed found a stronger reduction in the amplitude of EPSCs of the first as well as second pulses in recordings from knockout compared with wild-type mice ( Fig. 2 , first pulse WT: 0.45±0.02 versus KO: 0.38±002, P =0.008 and second pulse WT: 0.59±0.03 versus KO: 0.46±0.021; P =0.003, Student’s t -test, n =7 cells and three mice each). Our data are in line with the assumption that the absence of RIM1α leads to a reduction in P r , which in turn is reflected by a smaller glutamate transient in the synaptic cleft and therefore reduced displacement of γDGG from its receptors. As a control experiment, subsequent application of low concentrations of NBQX (200 nM) in contrast displayed similar depression of both EPSC responses in a paired-pulse stimulation protocol ( Fig. 2c , PPR wash=2.1±0.06 versus PPR in NBQX=2.2±0.09, not significant, one-way analysis of variance (ANOVA) with Bonferroni’s multiple comparison, n =5). 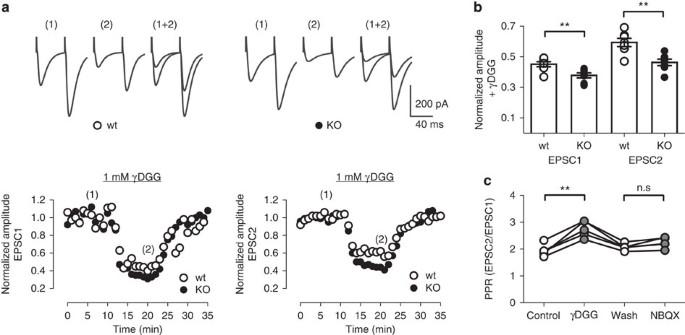Figure 2: Decreased synaptic glutamate transients in RIM1αknockout mice. 1 mM γDGG was applied for 10 min in order to receive relative estimates of the glutamate transient in the synaptic cleft. (a) Normalized amplitude is plotted over time for the first (left) and second (right) pulses of a 50-ms paired pulse. Data points shown are binned to 1 min. Top, example current traces for both genotypes taken at the time points indicated in the graphs below. (b) Summary bar graph for all experiments for the first and second pulses. Data points represent the average of the last 3 min before the washout of γDGG (n=7 each, bars report mean±s.e.m., **P<0.01, Student’st-test). (c) Summary graph depicting the effects of γDGG and NBQX on the paired-pulse ratio (PPR), measured in the same cells (n=5, **P<0.01 and n.s. not significant, one-way ANOVA with Bonferroni’s multiple comparison). Figure 2: Decreased synaptic glutamate transients in RIM1 α knockout mice. 1 mM γDGG was applied for 10 min in order to receive relative estimates of the glutamate transient in the synaptic cleft. ( a ) Normalized amplitude is plotted over time for the first (left) and second (right) pulses of a 50-ms paired pulse. Data points shown are binned to 1 min. Top, example current traces for both genotypes taken at the time points indicated in the graphs below. ( b ) Summary bar graph for all experiments for the first and second pulses. Data points represent the average of the last 3 min before the washout of γDGG ( n =7 each, bars report mean±s.e.m., ** P <0.01, Student’s t -test). ( c ) Summary graph depicting the effects of γDGG and NBQX on the paired-pulse ratio (PPR), measured in the same cells ( n =5, ** P <0.01 and n.s. not significant, one-way ANOVA with Bonferroni’s multiple comparison). Full size image Next, we performed a variance-mean analysis. Here EPSCs were recorded at five different external calcium concentrations and the variance was calculated from at least 30 samples at each epoch and plotted against the mean amplitude of the respective EPSC ( Fig. 3a–c ). We detected a significantly reduced P r in RIM1α −/− mice at concentrations from 2.5 to 4.5 mM calcium in comparison to responses from wild-type mice ( Fig. 3d , 2.5 mM Ca 2+ P r WT: 0.28±0.03, n =5 cells per four mice versus KO 0.14±0.03, n =5 cells per three mice; P =0.009 and 4.5 mM Ca 2+ WT: 0.66±0.04 versus KO 0.45±0.05; P =0.011, Student’s t -test). Both at the low (1 mM) and high end (5.5 mM) of concentrations tested ( Fig. 3d , 5.5 mM Ca 2+ , P r WT: 0.84±0.05 versus KO 0.77±0.05; P =0.36, Student’s t -test) no difference in P r was discernible between the two genotypes. The latter indicates that the release defect introduced by the deletion of RIM1α can be overcome by raising external calcium. In contrast, within a moderate range of calcium concentrations, deletion of RIM1α leads to a reduction in P r . The averaged quantal amplitude—that is, the response size to a released quantum—was similar in wild-type and RIM1α −/− mice ( Fig. 3e , Q av WT: 3.5±0.16 pA versus KO: 3.9±0.36 pA). 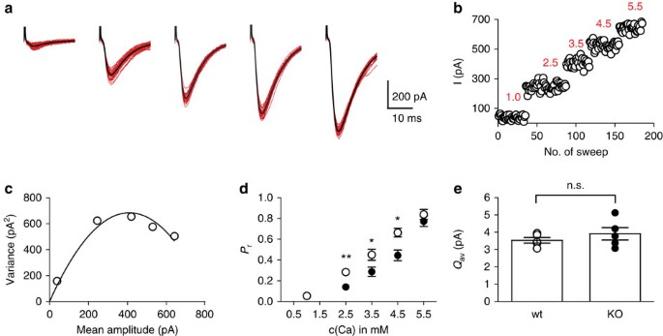Figure 3: Reduced release probability in the absence of RIM1α. Variance-mean analysis was performed to quantify differences in the functional synaptic properties of the granule cell—Purkinje cell synapse. (a–c) Representative example from a wild-type slice. (a) EPSCs were recorded under several differentPrconditions by altering Ca2+to Mg2+ratio. Single traces (red) and average (black) are shown for (from left to right in mM) 1.0, 2.5, 3.5, 4.5 and 5.5 Ca2+. (b) Plot of the analysed epochs. Red numbers indicate corresponding [Ca2+] in mM. The non-analysed epochs of the wash-in are left out for clarity. (c) Resulting variance-mean plot with respective points (circles) and fitted parabola (black line). Based on these curves, thePr(d) and averaged quantal content (Q) (e) were calculated for wild type (open circles,n=5) and RIM1α KO (filled circles,n=5); data are reported as mean±s.e.m., *P<0.05, **P<0.01 and n.s. not significant, Student’st-test. Figure 3: Reduced release probability in the absence of RIM1 α . Variance-mean analysis was performed to quantify differences in the functional synaptic properties of the granule cell—Purkinje cell synapse. ( a – c ) Representative example from a wild-type slice. ( a ) EPSCs were recorded under several different P r conditions by altering Ca 2+ to Mg 2+ ratio. Single traces (red) and average (black) are shown for (from left to right in mM) 1.0, 2.5, 3.5, 4.5 and 5.5 Ca 2+ . ( b ) Plot of the analysed epochs. Red numbers indicate corresponding [Ca 2+ ] in mM. The non-analysed epochs of the wash-in are left out for clarity. ( c ) Resulting variance-mean plot with respective points (circles) and fitted parabola (black line). Based on these curves, the P r ( d ) and averaged quantal content (Q) ( e ) were calculated for wild type (open circles, n =5) and RIM1α KO (filled circles, n =5); data are reported as mean±s.e.m., * P <0.05, ** P <0.01 and n.s. not significant, Student’s t -test. Full size image Reduced calcium influx in presynaptic boutons The obvious next question was by which mechanism RIM1α might affect P r ? Is it a direct function of RIM1α at the release machinery or rather an indirect process via interaction with VDCCs? To address this issue, we investigated whether RIM1α deletion affects calcium influx in the presynaptic granule cell axon terminals. Granule cells were patched and filled with a combination of two dyes, Alexa-594 (red channel) and Fluo4FF (green channel). At least 20 min after establishment of the whole-cell configuration lines, scans through individual granule cell boutons were recorded and both calcium-insensitive red signals as well as calcium responses (green signal) were recorded in epi- and transfluorescence pathways ( Fig. 4 ). In order to calculate the action potential-driven calcium influx into the terminals, we divided the green by the red signal and estimated the calcium concentration change according to established methods (refs 23 , 24 see methods ). We performed two sets of experiments; on one hand looking at boutons from the ascending segment (AA) of the granule cell axon and at the PF segment on the other. Those two segments have been described to have physiologically different properties and therefore should be distinguished [25] , [26] . Notably, the calculated peak calcium-influx change was considerably smaller in the terminals from RIM1α (−/−) than in wild-type mice both in boutons from the ascending axon and from the PF segment ( Fig. 4d,e , for PF: WT=0.31±0.02 μM, n =38 boutons per three mice versus KO=0.19±0.01 μM, n =35 boutons per three mice; P <0.001, and for AA: WT=0.42±0.03 μM, n =23 boutons per eight mice versus KO=0.31±0.02 μM, n =23 boutons per six mice, P =0.013, Student’s t -test). These data indicate a profound contribution of the RIM1α isoform to VDCC function or trafficking in presynaptic boutons of cerebellar granule cells. This reduction in calcium influx is most likely causal for the remarkable reduction in underlying P r and is reflected in altered STP behaviour in the absence of RIM1α. 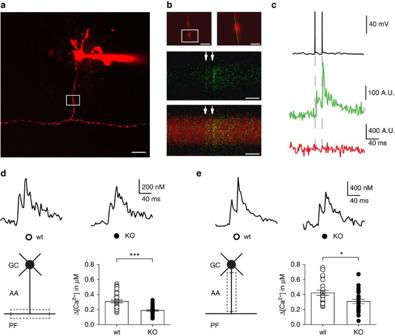Figure 4: Reduced presynaptic Ca2+influx in RIM1α-deficient mice. Two-photon laser-scanning fluorescence microscopy was used to assess the Ca2+transient at single boutons of the granule cell ascending axon and the parallel fibre segment. (a) Two-photon image of a cerebellar granule cell filled with Alexa-594 (30 μM) and fluo4FF (200 μM); scale bar=20 μm. (b) Medium (upper left, scale bar=2 μm) and high (upper right, scale bar=1 μm) magnification of a single ascending axon bouton. The yellow line indicates the orientation of the line scan (500 Hz) for the fluorescence measurement. Two action potentials (white arrows) with an interstimulus interval of 20 ms were elicited through current injection in the soma and the fluorescence intensity was recorded. The response to the paired action potentials is shown for the green channel (middle, scale bar=40 ms) and the green merged with the red channel (bottom, scale bar=40 ms). (c) Corresponding traces for the single trial shown in (b) of the somatic potential (top), the green channel (middle) and the red channel (bottom). (d) Representative calcium transients (average of four traces, binned to 250 Hz) for wild type and knockout and summary graph for both genotypes recorded from parallel fibre (PF) boutons. [Ca2+] changes are calculated from the average of four data points (16-ms interval) after the first peak. Bar graph shows average value and data points for individual boutons (open circle corresponds to WT, closed circles to KO); n(WT)=38, n(KO)=35, data are reported as mean±s.e.m., ***P<0.001. (e) Depicted are the recordings from boutons of the ascending axon with representative traces for each genotype (top) and summary graph (bottom);n=23 each, data are mean±s.e.m., *P<0.05, Student’st-test. Schematics on the left in (d) and (e) illustrate the location of recorded boutons from granule cell (GC) axons. Figure 4: Reduced presynaptic Ca 2+ influx in RIM1α-deficient mice. Two-photon laser-scanning fluorescence microscopy was used to assess the Ca 2+ transient at single boutons of the granule cell ascending axon and the parallel fibre segment. ( a ) Two-photon image of a cerebellar granule cell filled with Alexa-594 (30 μM) and fluo4FF (200 μM); scale bar=20 μm. ( b ) Medium (upper left, scale bar=2 μm) and high (upper right, scale bar=1 μm) magnification of a single ascending axon bouton. The yellow line indicates the orientation of the line scan (500 Hz) for the fluorescence measurement. Two action potentials (white arrows) with an interstimulus interval of 20 ms were elicited through current injection in the soma and the fluorescence intensity was recorded. The response to the paired action potentials is shown for the green channel (middle, scale bar=40 ms) and the green merged with the red channel (bottom, scale bar=40 ms). ( c ) Corresponding traces for the single trial shown in ( b ) of the somatic potential (top), the green channel (middle) and the red channel (bottom). ( d ) Representative calcium transients (average of four traces, binned to 250 Hz) for wild type and knockout and summary graph for both genotypes recorded from parallel fibre (PF) boutons. [Ca 2+ ] changes are calculated from the average of four data points (16-ms interval) after the first peak. Bar graph shows average value and data points for individual boutons (open circle corresponds to WT, closed circles to KO); n(WT)=38, n(KO)=35, data are reported as mean±s.e.m., *** P <0.001. ( e ) Depicted are the recordings from boutons of the ascending axon with representative traces for each genotype (top) and summary graph (bottom); n =23 each, data are mean±s.e.m., * P <0.05, Student’s t -test. Schematics on the left in ( d ) and ( e ) illustrate the location of recorded boutons from granule cell (GC) axons. Full size image Intact expression of long-term potentiation We finally wanted to explore the possible consequences that the reduced calcium influx in the absence of RIM1α might have on the induction and expression of presynaptic LTP at parallel-fibre synapses. The necessity of a rise in presynaptic terminal calcium for the induction of presynaptic LTP is well established [5] , and it is therefore conceivable that the observed reduction in calcium entry might lead to a failure of LTP induction. To begin with, we induced chemical LTP by application of 50 μM forskolin. In slices from both WT as well as RIM1α −/−, LTP was readily induced and expressed and showed no differences between the two genotypes ( Fig. 5a , WT 162.4±11.3%, n =9 slices, five mice versus KO 165.5±10.6%, n =9 slices, seven mice; P =0.84, Student’s t -test, values taken from averages of 26–30 min after induction). In the same lines, LTP induced by tetanic stimulation (8 Hz for 25 s) was also of the same magnitude in RIM1α −/− as observed in the wild-type condition ( Fig. 5b , WT 121.7±7.2%, n =8 slices, four mice versus KO 123.7±4.4%, n =7 slices, three mice; P =0.72, Student’s t -test, values taken from averages of 26–30 min after induction). Likewise, delivery of an induction protocol with a lesser number of total stimuli, 10 Hz for 10 s, that was used in previous publications, [11] resulted in a similar amount of potentiation in WT as well as RIM1α −/− slices ( Fig. 5c , WT 119.2±2.6, n =7 cells, five mice versus KO 118.6±7.5, n =8 cells, five mice, P =0.94, Student’s t -test). 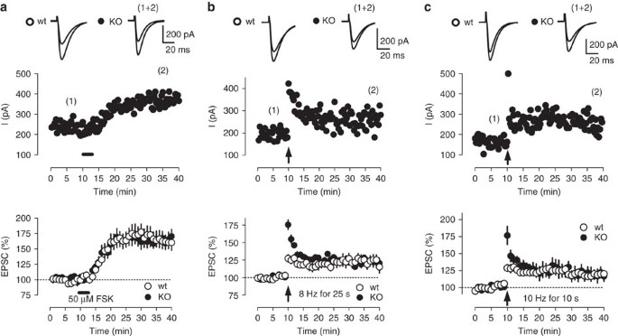Figure 5: Presynaptic long-term potentiation is unaltered in RIM1αknockout mice. LTP was induced by tetanic stimulation or chemically by application forskolin (a–c). (a) Application of forskolin (50 μM) for 3 min (bar);n=9 each. (b) Tetanic induction with 8 Hz for 25 s (arrow); n(WT)=8, n(KO)=7. (c) Tetanic stimulus protocol consisting of 10 Hz for 10 s (arrow); n(WT)=7, n(KO)=8. In each panel, on top are shown example traces for both genotypes, which represent the average of 5 min at the time points indicated in the graphs below. Middle shows the time course of a single experiment for RIM1a KO. Bottom displays summary data for WT (open circles) and KO (closed circles), in which values are plotted as mean±s.e.m. Figure 5: Presynaptic long-term potentiation is unaltered in RIM1 α knockout mice. LTP was induced by tetanic stimulation or chemically by application forskolin ( a – c ). ( a ) Application of forskolin (50 μM) for 3 min (bar); n =9 each. ( b ) Tetanic induction with 8 Hz for 25 s (arrow); n(WT)=8, n(KO)=7. ( c ) Tetanic stimulus protocol consisting of 10 Hz for 10 s (arrow); n(WT)=7, n(KO)=8. In each panel, on top are shown example traces for both genotypes, which represent the average of 5 min at the time points indicated in the graphs below. Middle shows the time course of a single experiment for RIM1a KO. Bottom displays summary data for WT (open circles) and KO (closed circles), in which values are plotted as mean±s.e.m. Full size image Of note in this latter set of experiments, there is a substantially stronger post-tetanic potentiation in RIM1α −/− slices, which can be observed with both tetanic-induction protocols. This fact again most likely reflects the reduced P r in the RIM1α −/− as compared with WT. From these data we conclude that the reduction in calcium entry in the absence of RIM1α does not lead to a failure of LTP induction and that this protein is not an absolute requirement for the expression of presynaptic LTP at the cerebellar PF synapses. In this report we describe the functional importance of RIM1α in setting the P r at the excitatory cerebellar PF synapse on the Purkinje neuron. We demonstrate that the absence of the single isoform RIM1α is sufficient to substantially reduce calcium influx in the granule cell axon terminals. Furthermore, as a functional consequence P r is decreased and STP is enhanced. In addition, we further show that loss of RIM1α does neither prevent induction nor expression of LTP, and therefore RIM1α is not an absolute requirement for the expression of LTP at this synapse. Two recent publications have demonstrated the role of RIM proteins in the targeting of VDCCs to presynaptic terminals. Loss of all RIM1/2 isoforms led to reductions in calcium current densities [18] and action potential evoked calcium transients measured with calcium-sensitive dyes [19] . An earlier study in expression systems had shown that RIM can also influence kinetic properties of calcium currents by reducing voltage-dependent inactivation [27] . Our results presented here show a robust reduction in calcium-influx amplitudes in granule cell boutons from mice lacking only the RIM1α isoform. Notably, we found a 30–40% calcium-influx reduction in the RIM1α KO, obviously already accounting for a large proportion of VDCC trafficking or functioning when compared with the 50% reduction in RIM1/2 KOs. The fact that the calcium-influx reduction in RIM1α −/− was somewhat smaller than those in the reports of Han et al . [18] and Kaeser et al . [19] might be explained by the fact that in our study only the RIM1α isoform was deleted, whereas in the other two studies all RIM1/2 isoforms were knocked out. The Calyx of Held synapse showed, in addition to reduced calcium currents, a modest decrease in P r and in turn displayed a reduced depression in response to stimulus trains in the absence of RIM 1 and 2 (ref. 18 ). The cortico-amygdala synapse is another preparation in which both a reduction in P r in combination with an increased STP has been described for RIM1α KOs [17] . The role of calcium influx was not tested in this latter study. The question remains whether the calcium-influx reduction that we find is responsible for the decrease in apparent P r ? From our data, assuming that calcium influx through VDCCs is only moderately saturated in the range of 1–5.5 mM external calcium concentration, one can see that a 30% reduction in external calcium. (3.5–2.5 mM) leads to some 40% reduction in P r in the wild-type situation (see Fig. 3d ). This value comes close to the reduction in P r ranging between 50 and 30% that we see in KO mice (over calcium concentrations from 2.5 to 4.5 mM), in which we found a decrease in calcium influx of roughly 30% in comparison with wild type. In addition, the deficit in P r in RIM1α KOs can be overcome by raising extracellular calcium concentration to higher levels (that is, 5.5 mM), where P r values reach the same magnitude as in the wild-type condition. Moreover, we also found smaller calcium transients in boutons from the PF segment of granule cells in comparison with boutons from the ascending axon segment ( Fig. 4d,e ). This observation corresponds well with a previous study by Sims and Hartell [25] demonstrating a smaller P r at synapses from the PF as compared with the ascending axon, further emphasizing the importance of calcium influx for P r . Therefore, our data indicate that calcium-influx reduction is a crucial factor for the reduced P r at the parallel fibre to Purkinje cell synapse. Furthermore, it is also very well conceivable that reductions in calcium influx may even lead to a complete shutdown of functional release sites (N) in RIM1α KO mice. In our variance-mean analysis approach, the number of release sites are primarily dependent on the amount of activated fibres, which is in turn set by the stimulation strength and position. As this cannot be adjusted with the desired precision between slices and genotypes, we had to refrain from calculating the parameter N. However, it remains an intriguing thought that the functional number of release sites could be reduced in RIM1α-deficient mice, and at the current stage we cannot exclude the possibility that the reduction in apparent P r may in part stem from a reduced number of functional release sites (N). However, VDCC targeting is seemingly not the only effect of RIMs that may result in reduced P r , as both the number of docked vesicles as well as the calcium sensitivity for transmitter release can be also affected by RIM deletion [18] . For this reason, further functional properties besides interaction with VDCCs of RIM proteins have also to be taken into consideration, which can additionally affect the reduction in P r besides reduced calcium influx. Those parameters could not be tested in the present study. Very likely it is a combination of all those factors acting in concert to set the P r ; however, RIM1α’s influence on VDCCs already seems to have a major impact on P r at the cerebellar parallel fibre synapse. In the majority of synapses tested so far, disruption of essential components of the priming or release apparatus has led to profound changes in the synapse STP behaviour (mostly meaning an increase in short-term facilitation), if transmission was not completely abolished. Such results have been described, for example, for complexins [28] , [29] , SV2 (refs 30 , 31 ), the RIM interaction partners Munc13s [32] , [33] and Rab3a [34] , as well as RIM1α itself [13] . In most of the reported cases, the STP changes were accompanied by or caused by a reduction in P r . A notable exception in this context is Rab3A, in which increased short-term facilitation was described with no alteration in P r at Schaffer-collateral synapses [13] , [34] . Only the complete deletion of all four Rab3 isoforms A–D was found to lead to reduced P r [15] , [35] . In the case of RIM1α and Rab3a, the situation was particularly special as their loss led to STP changes only in a synapse-specific manner: Increased short-term facilitation at the Schaffer collateral synapses [13] but unchanged STP at the hippocampal mossy fibre and cerebellar PF connections (in those latter cases they were essential for long-term potentiation instead) [11] . Our data instead add the PF synapse to the group of connections in which RIM1α deletion results in alterations of STP, which is explained by the described calcium-influx reduction. The currently held view on the mechanism of presynaptically expressed forms of LTP holds that RIM1α is an essential mediator in the expression of this process [5] , [22] , [36] , [37] . Two groups have found that in different preparations loss of RIM1α abolishes the expression of LTP at connections such as hippocampal mossy fibres, [11] cerebellar parallel fibres [11] and cortico-amygdala synapses [17] . Considering the recent data demonstrating the interaction of RIM1α with VDCCs and therefore presynaptic terminal calcium currents [18] , [19] , one could have speculated that the absence of LTP might be due to a failure of induction rather than expression because of insufficient calcium entry (even though this was taken into account in the original description of the LTP deficiency by raising extracellular calcium concentrations during induction, which was still not capable of rescuing LTP [11] ). However, in contrast we are able to show in this study that despite the absence of RIM1α, LTP can be induced normally at cerebellar PF synapses. These data challenge the view of RIM1α being an essential mediator of presynaptic LTP expression, but rather point to a role in altering the threshold for induction. The fact that PF-LTP can be readily obtained in conditions of reduced calcium entry is in line with other data in the literature. Pharmacologically blocking VDCCs responsible for presynaptic calcium entry such as P/Q-, N-type channels or reducing extracellular calcium concentration that reduce calcium influx to 20–50% did also not prevent the establishment of LTP at hippocampal mossy fibres [38] or cerebellar parallel fibres [39] . One possible explanation for the apparent discrepancy of our data with previously published results might be that a very subtle threshold level for LTP induction exists. This threshold could be sensitive to slight alterations in the level of extra- or intracellular calcium concentration or resting membrane potentials. The study of Myoga and Regehr [39] , for example, demonstrated that a small reduction of extracellular calcium from 1.5 to just 1.25 mM prevented the induction of LTP. In line with this latter finding we also found a loss of LTP in 1.25 mM external calcium, which is indicative of a rather sharp threshold for LTP induction. As for the chemical LTP induction with forskolin or cAMP analogues, there were already conflicting views in the literature whether or not in this situation RIM1α was necessary [11] , [40] . Moreover, mutation of a putative rotein kinase A (PKA) phosphorylation site on RIM1α was also found to not prevent presynaptic LTP [41] , casting additional doubt on the function of RIM1α as the ultimate target for presynaptic LTP expression. Whatever the underlying reason for the different results may be, our study might motivate further explorations into alternative molecular mechanisms of the expression of presynaptic LTP. Our results are more in line with a general and broad non-synapse-specific role of RIM in excitatory connections, in which its interaction with VDCCs ensures proper release and STP characteristics of synapses. Preparation of acute cerebellar tissue slices All experiments were carried out in accordance with the local and national guidelines (Berlin State Government, T0100/03). RIM1α KO mice and wild-type littermates of both sexes (3–6 weeks) were anesthetized and decapitated. The brain was quickly removed and cooled down in either low [Ca 2+ ] or (for Ca 2+ -imaging experiments) sucrose-based ACSF containing (in mM): 119 NaCl, 26 NaHCO 3 , 10 glucose, 2.5 KCl, 1 NaH 2 PO 4 , 0.5 CaCl 2 and 1.3 MgCl 2 or 87 NaCl, 26 NaHCO 3 , 50 sucrose, 10 glucose, 2.5 KCl, 1.25 NaH 2 PO 4 , 0.5 CaCl 2 and 3 MgCl 2 . Solutions were constantly oxygenated with carbogen (5% O 2 and 95% CO 2 ). Cerebellar slices (300 μm, sagittal or horizontal) were cut with a Leica VT1200S microtome (Wetzlar, Germany) and stored in the above solutions for 30 min at 35 °C. Subsequently, slices were stored in recording solution containing the following (in mM): 119 NaCl, 26 NaHCO 3 , 10 glucose, 2.5 KCl, 1 NaH 2 PO 4 , 2.5 CaCl 2 and 1.3 MgCl 2 at room temperature, and experiments were started after 30 min. Electrophysiological recordings Whole-cell recordings of Purkinje cells were carried out in the sagittal slices with a MultiClamp 700B (Axon Instruments, Union City, CA, USA) amplifier; signals were filtered at 2 kHz and digitized (National Instruments, BNC-2090) at 5 kHz, and recorded and analysed with custom-made software in IGOR Pro (WaveMetrics Inc., OR, USA). Experiments were performed in the presence of the GABA A receptor antagonist SR 95531 hydrobromide (1 μM). For recording borosilicate glass electrodes (2–5 MΩ) were filled with intracellular solution containing the following (in mM): 135 K-Gluconate, 20 KCl, 2 MgATP, 10 HEPES, 0.5 EGTA and 5 phosphocreatine. For extracellular fibre stimulation, a low-resistance patch pipette was filled with ACSF and placed in the molecular layer of the cerebellum, almost perpendicular to the Purkinje cell layer and the patched neuron. Stimulation frequency was 0.05 Hz or is mentioned in the text if otherwise. The tetanic-induction protocol for LTP consisted either of a 8-Hz train applied once for 25 s ( Fig. 5b ) or a 10-Hz train applied for 10 s ( Fig. 5c ). Chemical LTP was induced by applying forskolin at a concentration of 50 μM for 3 min. Recordings were carried out at room temperature. Series and input resistances (R s , R i ) were constantly monitored, and experiments were discarded if changes in the R s were >15%. Two-photon calcium imaging in granule cell boutons Two-photon Ca 2+ imaging was performed in horizontal slices at 34 °C. Granule cells were patched with thick-walled borosilicate glass electrodes (6–10 MΩ) filled with the following (in mM): 114 KMeSO 4 , 10 HEPES, 4 MgATP, 0.4 NaGTP and 14 phosphocreatine. The solution was complemented with 30 μM Alexa-594 for neuronal tracing and 200 μM Fluo4FF as intracellular Ca 2+ indicator. Pairs of action potentials for opening of VDCCs were evoked through current injection (250–600 pA) for 1 ms with an interstimulus interval of 20 ms. Experiments were started after 20 min of loading the cell with Alexa-594 and Fluo4FF to ensure a proper diffusion of the dyes and stable concentrations at the site of interest. Fluometric Ca 2+ measurements were performed with a two-photon laser-scanning system (Femto2D; Femtonics, Hungary) equipped with a femtosecond laser tuned to 805 or 810 nm (Chameleon; Coherent). Epifluorescence was collected with an Olympus LUMPlanFL N (60 × /1.0 NA) water-immersion objective, and for transfluorescence an Olympus oil-immersion condenser (1.4 NA) was used. Fluorescence was divided by a dichroic mirror at ~590–600 nm, and green and red signals were filtered using 525/50 and 650/50 bandpass filters, respectively. A diagram of the light path can be obtained from Chiovini et al . [42] Measurement control, data acquisition and analysis were performed using the Matlab-based MES program package (Femtonics). Line scans for fluometric measurements were performed with 500 Hz. In order to calculate Δ[Ca 2+ ] from the corresponding Δ G / R values, ( G / R ) min and ( G / R ) max were determined under conditions of 0 [Ca 2+ ] and saturating [Ca 2+ ] by adding 2 mM EGTA or 2 mM CaCl 2 to the pipette [23] , [43] . ( G / R ) max values under physiological conditions were validated by application of a 500-Hz train of APs for 1 s at the end of some experiments and similar ( G / R ) max ratios could be obtained. The procedure was repeated for all calcium-indicator stocks and wavelengths used. [Ca 2+ ] was then calculated according to the following equation with a K d =8.1 μM [23] : Data analysis and statistics To construct the variance-mean plot, EPSCs were recorded at five different release probabilities by altering Ca 2+ /Mg 2+ ratio. For every condition, epochs of at least 30 sweeps were chosen and controlled by a Spearman rank correlation test to fit the stability criterion. After subtraction of baseline noise variance, a simple parabola was fitted to the resulting variance-mean plot, which in all cases passed through a maximum. Experiments were excluded if the goodness of fit was R 2 <0.7. Weighted basal synaptic parameters ( P r , Q av ) were determined [44] , [45] according to the following equation: with and y =variance; mean amplitude; CV (Coefficient of variation of EPSC at individual release sites)=0.3. Statistical data analysis was performed using GraphPad Prism 5 (Graph Pad Software, La Jolla, USA). Results were considered significant if P <0.05 (* and ** for P <0.01) using an unpaired Student’s t -test, except for Fig. 2c , where a one-way ANOVA with Bonferroni’s multiple comparison was used. All numerical values are given as mean±s.e.m. Drugs and chemical compounds SR 95531 hydrobromide and γDGG were purchased from Tocris/Biozol (Eching, Germany), Alexa-594 and Fluo4FF from Invitrogen/Life Technologies (Darmstadt, Germany) and ACSF compounds from Roth (Karlsruhe, Germany). How to cite this article: Kintscher, M. et al . Role of RIM1α in short- and long-term synaptic plasticity at cerebellar parallel fibres. Nat. Commun. 4:2392 doi: 10.1038/ncomms3392 (2013).